Correspondence: Reply to ‘On the nature of strong piezoelectricity in graphene on SiO2’ 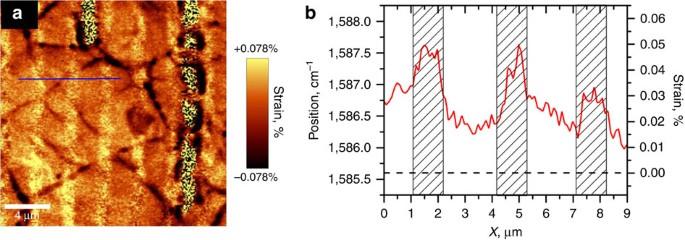Figure 1: Strains in the single-layer graphene on the silicon grating. (a) Strain map. (b) Variation of G-band position and strain across the grating (blue line ina); shaded rectangles correspond to supported graphene, dashed line denotes the initial (unstressed) value of G-band position. How to cite this article: da Cunha Rodrigues, G. et al . Correspondence: Reply to ‘On the nature of strong piezoelectricity in graphene on SiO 2 ’. Nat. Commun. 7:11571 doi: 10.1038/ncomms11571 (2016).